Microglia constitute a barrier that prevents neurotoxic protofibrillar Aβ42 hotspots around plaques In Alzheimer’s disease (AD), β-amyloid (Aβ) plaques are tightly enveloped by microglia processes, but the significance of this phenomenon is unknown. Here we show that microglia constitute a barrier with profound impact on plaque composition and toxicity. Using high-resolution confocal and in vivo two-photon imaging in AD mouse models, we demonstrate that this barrier prevents outward plaque expansion and leads to compact plaque microregions with low Aβ42 affinity. Areas uncovered by microglia are less compact but have high Aβ42 affinity, leading to the formation of protofibrillar Aβ42 hotspots that are associated with more severe axonal dystrophy. In ageing, microglia coverage is reduced leading to enlarged protofibrillar Aβ42 hotspots and more severe neuritic dystrophy. CX3CR1 gene deletion or anti-Aβ immunotherapy causes expansion of microglia coverage and reduced neuritic dystrophy. Failure of the microglia barrier and the accumulation of neurotoxic protofibrillar Aβ hotspots may constitute novel therapeutic and clinical imaging targets for AD. The mechanisms by which neural circuit disruption occurs in Alzheimer’s disease (AD) are not well understood. While genetic evidence in early-onset familial AD suggests a strong involvement of abnormal β-amyloid (Aβ) processing and aggregation [1] , in sporadic late-onset AD it is thought that disturbed Aβ clearance may lead to Aβ aggregation [2] , neuronal injury and dysfunction [3] . A variety of mechanisms of brain Aβ clearance have been postulated [4] , [5] , [6] including a role for microglia [7] , the resident immune and phagocytic cell in the central nervous system. The involvement of these cells in AD is further supported by recent studies showing that human genetic variants in microglia-related molecules, such as TREM2 and C D33 are associated with an increased risk of late-onset AD [8] , [9] , [10] , [11] , [12] . Microglia are highly motile cells that constantly survey the brain microenvironment and undergo activation in response to a diverse range of tissue perturbations [13] , [14] . One striking feature of the behaviour of microglia in the AD brain is their marked clustering around fibrillar Aβ deposits, which are also in close proximity to dendrites with reduced spine density and dystrophic axons [15] , [16] , [17] , [18] , [19] . Plaque-associated microglia display an activated and polarized morphology with their processes pointed towards and highly intertwined with the plaque surface [16] , [20] , [21] . Despite this close interaction, in vivo mouse data have shown that microglia are very ineffective at phagocytosis of fibrillar amyloid deposits [16] , [19] , [22] but are instead able to take up prefibrillar forms of Aβ [7] , [19] . In addition, modulation of microglia-related chemokine receptors or anti-Aβ immunization, both of which can affect microglia activation status, have been shown to influence the degree of brain amyloid accumulation [18] , [19] , [23] , [24] , [25] , [26] , [27] , [28] , [29] , [30] . While these effects on amyloid burden may partly be explained by Aβ phagocytosis [19] , microglia could possess additional unknown functions that may affect the evolution of amyloid deposition. Furthermore, due to their close proximity to axonal structures and their potential for producing neurotoxic cytokines and reactive oxygen species [31] , some suggest that microglia play a causative role in the formation of dystrophic neurites. On the other hand, microglia could play neuroprotective roles through mechanisms not yet identified [32] . Thus, it remains unknown whether the aspects of microglia function play beneficial or detrimental roles that could be specifically targeted for therapeutic purposes. To address this gap in knowledge, we developed in vivo methods using two-photon and high-resolution confocal microscopy for examining the role of microglia in the dynamic equilibrium between soluble interstitial Aβ and fibrillar amyloid deposits, amyloid plaque expansion and the resulting toxicity to adjacent neurons. Our data reveal a striking pattern of anti-co-localization between microglia processes, protofibrillar Aβ42 and dystrophic axons. We demonstrate that this pattern is due to microglia acting as a barrier that restricts the radial expansion of plaques by controlling their affinity for soluble Aβ, a function that we show is critical for limiting the formation of neurotoxic hotspots of protofibrillar Aβ42 around plaques. Modulation of microglia activity by either CX3CR1 receptor deletion or passive anti-Aβ immunization leads to the expansion of the microglia barrier with a consequent reduction in plaque neurotoxicity. Finally, we show that certain natural and synthetic small molecules have the ability to selectively target these neurotoxic protofibrillar Aβ42 hotspots, raising the possibility that analogous compounds could be used therapeutically or in clinical imaging applications. Microglia plaque envelopment does not prevent diffusion of soluble Aβ into the plaque core We first quantified the extent to which the surface of individual amyloid plaques was covered by the processes of adjacent microglia in two Alzheimer-like transgenic mouse models (5xFAD and CRND8). In our analysis of confocal image stacks of brain slices with labelled microglia and fibrillar amyloid plaques, we observed that larger plaques tended to have less microglia coverage than smaller ones, but overall there was a great heterogeneity in the degree of microglia coverage ( Fig. 1a,b ). Given that microglial processes are known to be highly motile in the normal brain [13] , we next asked how physically stable the processes involved in tightly wrapping plaques were compared with those that did not contact plaques. To address this, we used in vivo two-photon imaging to visualize plaques and microglia in 5 × FAD mice expressing green fluorescent protein (GFP) exclusively in microglia. We found that over intervals of minutes to days, the microglial processes wrapping plaques were highly stable in contrast to the motile processes in the same cells that were not contacting plaques ( Fig. 1c–g and Supplementary Movie 1 ). However, when we monitored the same individual plaques and microglia over intervals of months, we observed some rearrangement of the microglia processes contacting plaques, with an overall significant reduction in the degree of coverage ( Fig. 1e–g ), consistent with our data from fixed tissues showing that the degree of microglial coverage is lower as plaques grow in size ( Fig. 1b ). 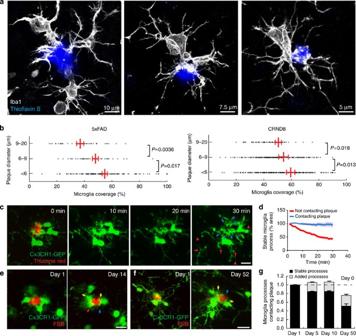Figure 1: Microglia process envelopment of plaques is stable over weeksin vivo. (a) Representative confocal images of Iba1 immunolabelled microglia around Thioflavin S-labelled amyloid plaques in a 4-month-old 5 × FAD mouse. (b) Quantification of microglia coverage in 4-month-old 5 × FAD and 4-month-old CRND8 mice. Microglia coverage was quantified as the percentage of plaque perimeter contacted by microglia process.N>90 plaques (1–20 μm in diameter) from five animals for each transgenic line. Red bars represent mean±s.e.m. (unpairedt-test,t=(84)2.998 and(156)2.422 in 5 × FAD andt=(218)2.379 and(362)2.506 in CRND8). (c)In vivotime-lapse images of the microglia around amyloid plaques inCX3CR1-GFP × 5 × FAD mouse. Blue arrows: microglia processes contacting amyloid plaques; red arrows: processes not in contact with amyloid plaque and extended between 20th and 30th min of the imaging session; red arrowheads: processes not in contact with amyloid plaque and regressed between 20th and 30th min of the imaging session. (d) Quantification of microglia process stability over 30 min.N=15 plaques in five animals. Data represent mean s.e.m. (e,f).In vivotime-lapse imaging over weeks to months reveals the stability of microglia processes contacting amyloid plaques. Stable processes: yellow arrows; newly added processes: red arrows; regressed processes: blue arrows. (g) Quantification of long-term dynamism of microglia processes contacting amyloid plaques.N=51 plaques in nine animals. Scale bars, 5 μm inc,eandf. Figure 1: Microglia process envelopment of plaques is stable over weeks in vivo . ( a ) Representative confocal images of Iba1 immunolabelled microglia around Thioflavin S-labelled amyloid plaques in a 4-month-old 5 × FAD mouse. ( b ) Quantification of microglia coverage in 4-month-old 5 × FAD and 4-month-old CRND8 mice. Microglia coverage was quantified as the percentage of plaque perimeter contacted by microglia process. N >90 plaques (1–20 μm in diameter) from five animals for each transgenic line. Red bars represent mean±s.e.m. (unpaired t- test, t = (84) 2.998 and (156) 2.422 in 5 × FAD and t = (218) 2.379 and (362) 2.506 in CRND8). ( c ) In vivo time-lapse images of the microglia around amyloid plaques in CX3CR1 -GFP × 5 × FAD mouse. Blue arrows: microglia processes contacting amyloid plaques; red arrows: processes not in contact with amyloid plaque and extended between 20th and 30th min of the imaging session; red arrowheads: processes not in contact with amyloid plaque and regressed between 20th and 30th min of the imaging session. ( d ) Quantification of microglia process stability over 30 min. N =15 plaques in five animals. Data represent mean s.e.m. ( e , f ). In vivo time-lapse imaging over weeks to months reveals the stability of microglia processes contacting amyloid plaques. Stable processes: yellow arrows; newly added processes: red arrows; regressed processes: blue arrows. ( g ) Quantification of long-term dynamism of microglia processes contacting amyloid plaques. N =51 plaques in nine animals. Scale bars, 5 μm in c , e and f . Full size image Given the tight and stable contact between microglia processes with the plaque surface [22] , we asked whether this interaction was capable of restricting the binding of interstitial soluble Aβ to the plaque. We performed in vivo two-photon imaging of fibrillar amyloid plaques prelabelled with the fluorescent fibrillar amyloid-binding dye (E,E)-1-fluoro-2,5-bis(3-hydroxycarbonyl-4-hydroxy)styrylbenzene (FSB), while simultaneously microinjecting fluorescently conjugated soluble Aβ40-555 or Aβ42-555 into the subarachnoid space ( Fig. 2a,b ). Within minutes of injection, both Aβ40 and Aβ42 are diffused throughout the hemisphere and rapidly bound with high-affinity to pre-existing FSB-labelled fibrillar plaques ( Fig. 2c–e and Supplementary Movie 2 ). Thus, even among the most robustly enveloped amyloid plaques, microglia processes are not capable of preventing the diffusion of Aβ into the plaque core. 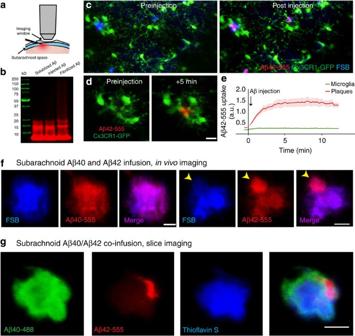Figure 2:In vivobrain infusion reveals hotspots of Aβ42 binding to existing plaques. (a) Hylite-555 labelled-Aβ40 or Aβ42 was infused into the mouse brain via the subarachnoid space and imaged through a thinned-skull window away from the injection site. (b) SDS–PAGE analysis of the soluble Aβ42 used forin vivoinfusion andex vivobrain slice labelling. Fluorescently labelled Aβ42 stock solution (DMSO, 1 μg μl−1) was diluted in ACSF (1:9 v/v) on ice. Three different preparations of Aβ42 were analysed using SDS–PAGE gel. The SDS–PAGE analysis indicated that the main Aβ species injected were monomers and small oligomers. (c,d)In vivotwo-photon time-lapse images inCX3CR1/5 × FAD mice show that Aβ42-555 (red) rapidly binds to the existing amyloid plaques, prelabelled by FSB (blue) that are extensively surrounded by microglia (green). (e) Quantification of Aβ42-555 fluorescence during injection. Aβ42-555 binds to the pre-existing amyloid plaque rapidly and with very high specificity. Internalization by surrounding microglia was undetectable in this time frame.N=30 plaques in five animals. Data represents mean±s.e.m. (f) High magnification two-photon images show hotspots of Aβ42-555 binding to amyloid plaques (arrowhead). In contrast Aβ40-555 infusions led to homogeneous binding to amyloid plaques. (g) Simultaneousin vivoinfusion of Aβ42-555 and Aβ40-488 followed by confocal imaging in the fixed slices. Figure 2: In vivo brain infusion reveals hotspots of Aβ42 binding to existing plaques. ( a ) Hylite-555 labelled-Aβ40 or Aβ42 was infused into the mouse brain via the subarachnoid space and imaged through a thinned-skull window away from the injection site. ( b ) SDS–PAGE analysis of the soluble Aβ42 used for in vivo infusion and ex vivo brain slice labelling. Fluorescently labelled Aβ42 stock solution (DMSO, 1 μg μl −1 ) was diluted in ACSF (1:9 v/v) on ice. Three different preparations of Aβ42 were analysed using SDS–PAGE gel. The SDS–PAGE analysis indicated that the main Aβ species injected were monomers and small oligomers. ( c , d ) In vivo two-photon time-lapse images in CX3CR1 /5 × FAD mice show that Aβ42-555 (red) rapidly binds to the existing amyloid plaques, prelabelled by FSB (blue) that are extensively surrounded by microglia (green). ( e ) Quantification of Aβ42-555 fluorescence during injection. Aβ42-555 binds to the pre-existing amyloid plaque rapidly and with very high specificity. Internalization by surrounding microglia was undetectable in this time frame. N =30 plaques in five animals. Data represents mean±s.e.m. ( f ) High magnification two-photon images show hotspots of Aβ42-555 binding to amyloid plaques (arrowhead). In contrast Aβ40-555 infusions led to homogeneous binding to amyloid plaques. ( g ) Simultaneous in vivo infusion of Aβ42-555 and Aβ40-488 followed by confocal imaging in the fixed slices. Full size image Soluble Aβ42 has a high affinity for plaque microregions with low fibrillar amyloid density We then imaged plaques at a higher resolution after subarachnoid Aβ-555 infusion and were surprised to observe a striking difference between Aβ40 and Aβ42. Aβ42-555 showed a very heterogeneous binding pattern with hotspots of markedly increased affinity ( Fig. 2f ), while Aβ40-555 binding was more homogeneous throughout the plaque ( Fig. 2f,g , Supplementary Fig. 1a ). The dramatic discrepancy in binding patterns is unlikely to be due to the differential diffusion properties of Aβ40 and Aβ42 given their similar molecular size and the fact that an identical pattern of Aβ42 hotspot binding was observed after directly exposing plaques to Aβ42 in either unfixed freshly cut or fixed and permeabilized brain slices ( Fig. 3a,b ). Furthermore, a scrambled Aβ42 peptide did not bind to the plaques at all ( Supplementary Fig. 1c ). Importantly, immunohistochemistry on fixed brain slices with C-terminal specific antibodies demonstrated that endogenous Aβ42 also accumulates in these hotspot microregions ( Fig. 3c ). This strongly suggests that plaque microregions have distinct biochemical conformations that cause differential and specific Aβ42 affinities leading to the observed hotspots. 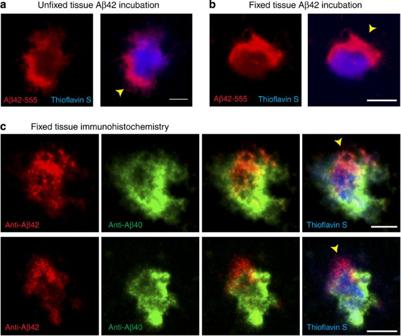Figure 3: Endogenous Aβ42 accumulates within plaque hotspotsin vivo. (a,b) Representative confocal images show hotspots of Aβ42-555 binding (arrowheads) in fresh unfixed (a) and fixed-permeabilized brain slices (b). (c) Immunohistochemistry with Aβ42 and Aβ40 C-terminus specific antibodies on fixed brain slices from mice that did not receive an Aβ-555 injections. Scale bars, 5 μm in all panels. Figure 3: Endogenous Aβ42 accumulates within plaque hotspots in vivo . ( a , b ) Representative confocal images show hotspots of Aβ42-555 binding (arrowheads) in fresh unfixed ( a ) and fixed-permeabilized brain slices ( b ). ( c ) Immunohistochemistry with Aβ42 and Aβ40 C-terminus specific antibodies on fixed brain slices from mice that did not receive an Aβ-555 injections. Scale bars, 5 μm in all panels. Full size image We further examined the intrinsic differences between plaque microregions with or without Aβ42-555 hotspots ( Fig. 4a ). We found that Aβ42 hotspots invariably colocalized with regions containing low fibrillar amyloid density, as evidenced by the inverse relationship between Aβ42 and Thioflavin S (TS) fluorescence intensities ( Fig. 4b–e ). Furthermore, non-hotspot areas were characterized by a more distinct TS-labelled fibrillar plaque edge, compared with the gradual tapering of TS labelling near Aβ42 hotspots ( Fig. 4f–h ). This indicates that the presence of pre-existing amyloid fibrils is critical for the soluble Aβ42 binding to occur, but as the amyloid plaque becomes gradually denser and compact, the affinity for new soluble Aβ42 is dramatically reduced. 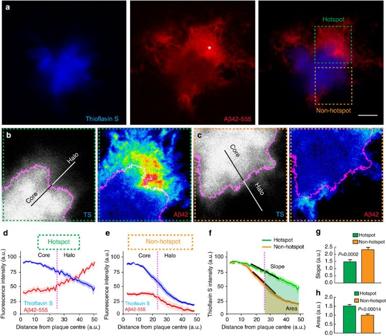Figure 4: Aβ42 hotspots occur in distinct plaque regions with sparse fibrillar amyloid. (a) Representative confocal images of Aβ42-555 binding to fibrillar amyloid plaque (asterisk indicates a prominent Aβ42 hotspot). Scale bar, 5 μm. Dashed squares point to areas with (green) and without (orange) an Aβ42 hotspot. (b,c) Intensity (heat) maps of plaque borders pointing towards a hotspot (b) and a non-hotspot (c) area, depicted at low zoom ina. The magenta outline inbandcrepresents the thresholded plaque border separating the plaque core from the halo. (d,e) Line profiles of fluorescence intensities across the plaque borders (magenta dotted lines) as shown inbandc. Data represents mean±s.e.m. (f–h) Quantification of thioflavin S fluorescence change as a function of distance from the plaque centre in the hotspot and non-hotspot areas. The slope of the curves indicates the rate of fluorescence change (how compact are the fibrils at the plaque edge) and the area under the curve represents the amount of fibrillar amyloid (total TS fluorescence) in the plaque halo area. Data represents mean±s.e.m. (unpairedt-test,t=(47)4.005 ing,t=(34)4.299 inh). Ford–hN=30 plaques with diameter <10 μm from 2 5 × FAD mice (6 months old). Figure 4: Aβ42 hotspots occur in distinct plaque regions with sparse fibrillar amyloid. ( a ) Representative confocal images of Aβ42-555 binding to fibrillar amyloid plaque (asterisk indicates a prominent Aβ42 hotspot). Scale bar, 5 μm. Dashed squares point to areas with (green) and without (orange) an Aβ42 hotspot. ( b , c ) Intensity (heat) maps of plaque borders pointing towards a hotspot ( b ) and a non-hotspot ( c ) area, depicted at low zoom in a . The magenta outline in b and c represents the thresholded plaque border separating the plaque core from the halo. ( d , e ) Line profiles of fluorescence intensities across the plaque borders (magenta dotted lines) as shown in b and c . Data represents mean±s.e.m. ( f – h ) Quantification of thioflavin S fluorescence change as a function of distance from the plaque centre in the hotspot and non-hotspot areas. The slope of the curves indicates the rate of fluorescence change (how compact are the fibrils at the plaque edge) and the area under the curve represents the amount of fibrillar amyloid (total TS fluorescence) in the plaque halo area. Data represents mean±s.e.m. (unpaired t -test, t = (47) 4.005 in g , t = (34) 4.299 in h ). For d – h N =30 plaques with diameter <10 μm from 2 5 × FAD mice (6 months old). Full size image Aβ42 hotspots are anti-co-localized with microglia processes Given the incomplete plaque coverage by microglia ( Fig. 1 ), we next explored the possibility that the patchy fibrillar plaque affinity for soluble Aβ42 is influenced by the presence of microglia processes. To examine this, we obtained high-resolution confocal images of microglia around plaques and correlated their location with the presence of Aβ42-555 hotspots and the relative density of fibrillar amyloid (TS fluorescence). We found that plaque surface regions not covered by microglia processes had a much lower TS fluorescence intensity ( Supplementary Fig. 3 ) but exhibited strong Aβ42-555 labelling, while immediately adjacent regions wrapped by microglia processes had greater TS fluorescence but much less Aβ42-555 labelling ( Fig. 5a–c ). Furthermore, smaller plaques that tended to be completely wrapped by microglia processes and had minimal Aβ42 binding, while larger plaques were less covered by microglia but showed high-affinity Aβ42 binding ( Fig. 5d,e ). 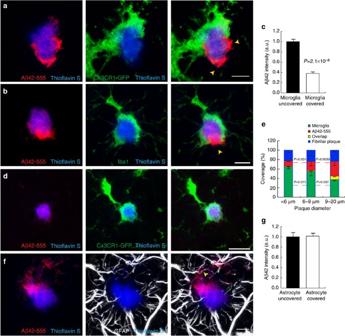Figure 5: Microglia but not astrocyte processes are anti-co-localized with Aβ42 hotspots. (a,b) Representative confocal images of Aβ42 hotspot (arrowheads) and surrounding microglia. Microglia were labelled by crossbreeding withCX3CR1-GFP mice. (b) Quantification of Aβ42-555 fluorescence in areas covered or uncovered by the microglia.N=60 plaques from three mice. Data represents mean±s.e.m. (unpairedt-test,t=(58)6.309). (c–e) Microglia coverage decreases as plaques grow while Aβ42 hotspot becomes more prominent. Small plaques tend to be completely wrapped by microglia without hotspot (d). Quantification of plaque perimeters in different size groups show that plaque size negatively correlated with microglia coverage, while positively correlated with Aβ42 hotspot (e).N=60 plaques from three mice. Data represents mean±s.e.m; the corresponding groups in each plaque size bin were compared with unpairedt-test (t=(30)2.728 and(22)2.218 for microglia coverage.t=(30)2.253 and(22)3.223 for Aβ42 coverage). (f,g) Astrocytic processes (labelled with GFAP (glial fibrillary acidic protein)) around amyloid plaques do not correlate with Aβ42 hotspot.N=60 plaques from three mice. Data represents mean±s.e.m. Scale bars, 5 μm in all panels. Figure 5: Microglia but not astrocyte processes are anti-co-localized with Aβ42 hotspots. ( a , b ) Representative confocal images of Aβ42 hotspot (arrowheads) and surrounding microglia. Microglia were labelled by crossbreeding with CX3CR1 -GFP mice. ( b ) Quantification of Aβ42-555 fluorescence in areas covered or uncovered by the microglia. N =60 plaques from three mice. Data represents mean±s.e.m. (unpaired t -test, t = (58) 6.309). ( c – e ) Microglia coverage decreases as plaques grow while Aβ42 hotspot becomes more prominent. Small plaques tend to be completely wrapped by microglia without hotspot ( d ). Quantification of plaque perimeters in different size groups show that plaque size negatively correlated with microglia coverage, while positively correlated with Aβ42 hotspot ( e ). N =60 plaques from three mice. Data represents mean±s.e.m; the corresponding groups in each plaque size bin were compared with unpaired t -test ( t = (30) 2.728 and (22) 2.218 for microglia coverage. t = (30) 2.253 and (22) 3.223 for Aβ42 coverage). ( f , g ) Astrocytic processes (labelled with GFAP (glial fibrillary acidic protein)) around amyloid plaques do not correlate with Aβ42 hotspot. N =60 plaques from three mice. Data represents mean±s.e.m. Scale bars, 5 μm in all panels. Full size image In contrast to microglia, the location of reactive astrocytes, which also have polarized processes making extensive contact with the plaque surface, did not show any spatial correlation with TS or Aβ42-555 fluorescence ( Fig. 5f,g and Supplementary Fig. 5 ). Thus, these data strongly suggest that the presence of microglial processes is a critical determinant of the degree of amyloid compaction, which markedly affects the affinity of plaques to soluble Aβ42. Protofibrillar Aβ42 hotspots can be revealed with specific Aβ binding dyes Given our findings that plaque microregions with low levels of amyloid compaction in microglia-uncovered areas have a much greater affinity for exogenous Aβ42-555, we hypothesized that these areas would also be sites of active binding and polymerization of endogenously produced Aβ. However, endogenous forms of protofibrillar Aβ are difficult to visualize in intact tissues because of a lack of specific antibodies for these Aβ conformations. Instead, we tested the properties of a variety of fluorescent small molecule dyes known to have affinity for amyloid plaques. We found that like Thioflavin S, the majority of Congo red and Thioflavin-T derivatives mainly bind to the fibrillar plaque core ( Fig. 6c–h ). Surprisingly, the natural product Curcumin [33] and the synthetic compound THK-265 [34] both displayed a unique binding pattern remarkably similar to that of exogenously infused Aβ42 ( Fig. 6a,b,i and Supplementary Fig. 1e ). Curcumin has been shown in vitro to bind oligomeric and protofibrillar Aβ [33] , [35] . To determine whether Curcumin and THK-265 are binding to oligomeric Aβ enriched in these hotspots, we immunolabelled brain slices with the oligomer-specific antibodies A11 and OC [36] , [37] . These antibodies, however, did not show any hotspot pattern, but instead labelled the plaque perimeters uniformly as well as small puncta throughout the brain parenchyma ( Supplementary Fig. 2 ), suggesting that hotspots are not enriched in Aβ oligomers. The fact that the labelling by Curcumin and THK-265 but not TS is highly co-localized with that of infused Aβ42-555 and endogenous Aβ42 immunolabelling ( Fig. 3c ), strongly suggests that hotspots are sites of active aggregation for endogenous Aβ42 into protofibrils. 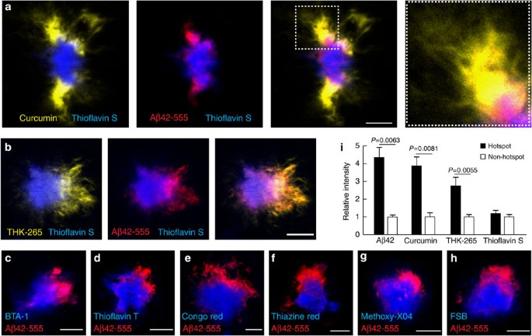Figure 6: Unique plaque-labelling patterns of Aβ binding dyes. (a–h) Representative confocal images in fixed slices demonstrate unique labelling patterns for various β-sheet binding dyes.In vivosubarachnoid infusion of Aβ42-555 (red) was performed 1 day before slice dye labelling. Scale bars, 5 μm. (i) Quantification of different β-sheet binding dyes labelling in Aβ42-555 hotspot and non-hotspot areas.N>10 plaques for each dye. Data represents mean±s.e.m. (unpairedt-test,t=(14)3.210,(14)3.090 and(15)2.900). Figure 6: Unique plaque-labelling patterns of Aβ binding dyes. ( a – h ) Representative confocal images in fixed slices demonstrate unique labelling patterns for various β-sheet binding dyes. In vivo subarachnoid infusion of Aβ42-555 (red) was performed 1 day before slice dye labelling. Scale bars, 5 μm. ( i ) Quantification of different β-sheet binding dyes labelling in Aβ42-555 hotspot and non-hotspot areas. N >10 plaques for each dye. Data represents mean±s.e.m. (unpaired t -test, t = (14) 3.210, (14) 3.090 and (15) 2.900). Full size image These data demonstrate that the protofibrillar Aβ42 hotspots are determined by intrinsic biochemical differences within plaque microregions that can be unambiguously revealed in vivo by fluorescently labelled Aβ42 or specific Aβ binding dyes. Neuritic dystrophy is more severe next to plaque regions lacking microglia processes Oligomeric and protofibrillar forms of Aβ have been shown to be significantly more neurotoxic than larger Aβ aggregates [38] , [39] . Given our finding that plaque microregions not covered by microglia, are hotspots rich in protofibrillar Aβ42, we asked whether these regions were associated with greater axonal dystrophy than the adjacent ones that were covered by microglia processes. To address this question, we first performed immunolabelling of dystrophic neurites using anti-Lamp1 or anti-Ubiquitin antibodies, which robustly demarcate the swollen dystrophic axons around fibrillar amyloid plaques as previously shown by confocal [40] and electron microscopy [41] , [42] , [43] ( Fig. 7a–d ). Quantitative confocal microscopy revealed that plaque regions covered by microglia had significantly fewer dystrophic neurites than those without microglia processes ( Fig. 7b,d ). We then examined the dynamics of dystrophic neurite (DN) formation and elimination by in vivo two-photon imaging and correlated it with the location of microglia processes. We used a triple transgenic strategy by crossbreeding 5 × FAD mice with mice expressing GFP in microglia ( CX3CR1 GFP/+ ), while neurons were labelled by further crossbreeding with mice expressing yellow fluorescent protein (YFP) under the Thy1 promoter or by cortical infection with an adeno-associated virus driving neuronal expression of tdTomato. We found that areas not covered by microglia had an even greater degree of axonal dystrophy than microglia-covered areas compared with what was apparent by anti-Lamp1 or anti-Ubiquitin immunolabelling ( Fig. 7e,f ). Furthermore, time-lapse in vivo imaging showed a markedly increased rate of DN formation in areas lacking microglia processes ( Fig. 7g,h ), supporting the concept of increased neurotoxicity by protofibrillar Aβ42 hotspots. 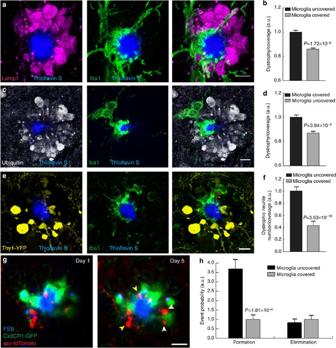Figure 7: Microglia processes protect adjacent neurites from protofibrillar Aβ42 toxicity. (a–d) Representative confocal image analysis of the degree of microglia coverage (Iba1, green) versus extent of neuritic dystrophy (Lamp1, magenta or Ubiquitin, grey). Graphs inb,drepresent the area of dystrophic neurites extending radially outward from microglia-covered or -uncovered plaque perimeter. The degree of neuritic dystrophy (yaxis) is normalized by the angular plaque coverage by microglia processes (see Methods for detail).N>60 plaques from three mice. Data represents mean±s.e.m. (pairedt-test,t=(57)4.694 inaand(67)4.410 forb). (e,f) Representative confocal images of microglia and dystrophic neurites around amyloid plaques in Thy1-YFP/5 × FAD mice. Quantification of DN number was done as inbandd.N=70 plaques from four mice. Data represents mean±s.e.m. (pairedt-test,t=(67)8.290). (g,h) Two-photon transcranialin vivotime-lapse images of DN dynamics around amyloid plaques. Newly formed (white arrowhead) and stable (yellow arrowhead) dystrophic neurites (labelled in either Thy1-YFP mice or by AAV-TdTomato injections) were quantified (data are a combination of both labelling methods). Data comes from eight mice and 45 plaques. Data represents mean±s.e.m. (pairedt-test,t=(42)4.108). Scale bars, 5 μm in all panels. Figure 7: Microglia processes protect adjacent neurites from protofibrillar Aβ42 toxicity. ( a–d ) Representative confocal image analysis of the degree of microglia coverage (Iba1, green) versus extent of neuritic dystrophy (Lamp1, magenta or Ubiquitin, grey). Graphs in b , d represent the area of dystrophic neurites extending radially outward from microglia-covered or -uncovered plaque perimeter. The degree of neuritic dystrophy ( y axis) is normalized by the angular plaque coverage by microglia processes (see Methods for detail). N >60 plaques from three mice. Data represents mean±s.e.m. (paired t -test, t = (57) 4.694 in a and (67) 4.410 for b ). ( e , f ) Representative confocal images of microglia and dystrophic neurites around amyloid plaques in Thy1-YFP/5 × FAD mice. Quantification of DN number was done as in b and d . N =70 plaques from four mice. Data represents mean±s.e.m. (paired t -test, t = (67) 8.290). ( g , h ) Two-photon transcranial in vivo time-lapse images of DN dynamics around amyloid plaques. Newly formed (white arrowhead) and stable (yellow arrowhead) dystrophic neurites (labelled in either Thy1-YFP mice or by AAV-TdTomato injections) were quantified (data are a combination of both labelling methods). Data comes from eight mice and 45 plaques. Data represents mean±s.e.m. (paired t -test, t = (42) 4.108). Scale bars, 5 μm in all panels. Full size image Taken together, these data demonstrate that plaque areas without microglia processes are sites of greater neurotoxicity likely due to the accumulation of endogenous protofibrillar Aβ42. Furthermore, it suggests that microglia act as a barrier that shields neurons from the local toxicity associated with the ongoing aggregation of Aβ. The neuroprotective barrier provided by microglia declines in ageing To explore the effects of ageing on the ability of microglia to form an effective barrier, we compared the number of microglia and their degree of coverage of the plaque surface across different ages. We found that as mice became older there was a gradual decrease in the average number of microglia within a 25-μm radius of the plaque perimeter ( Fig. 8a ), which was at least partly due to a diminished proliferative capacity ( Fig. 8b ). This reduction led to a significant difference in the degree of microglia process envelopment of the plaque surface ( Fig. 8a ). We then probed whether this microglia reduction had any effect on the degree of Aβ aggregation and toxicity around plaques. We first looked at the amount of protofibrillar Aβ42 by measuring the perimeter of curcumin labelling around the plaques of various sizes and at different mouse ages. Interestingly, we found that in 18 to 24 month-old CRND8 mice, plaques of equivalent size as in 4–month–old mice had a markedly increased protofibrillar Aβ42 halo ( Fig. 8c,e and Supplementary Fig. 8 ). Furthermore, the accumulation of protofibrillar Aβ was associated with a large increase in the area of dystrophic neurites ( Fig. 8d,f ). These data demonstrate that microglia ageing is associated with a profound increase in the accumulation of protofibrillar Aβ around plaques and in worsened neuritic pathology, which could be partly due to an ineffective microglia barrier function. 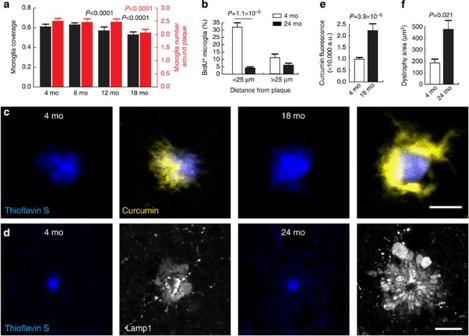Figure 8: Reduced microglia coverage in ageing is associated with an increased Aβ halo and neurotoxicity. (a) Quantification of microglia coverage (black bars) and microglia number (red bars) within 25 μm from the plaque edge at different ages in CRND8 mice.N>120 plaques from four mice per age group. Data represents mean±s.e.m. (unpairedt-test,t=(373)3.905 and(286)5.602 in microglia coverage andt=(286)3.325 in microglia number). (b) Quantification of BrdU+ (5-bromodeoxyuridine ) microglia in 4 and 24 month-CRND8 mice. N=222 and 100 field of views analysed for 24 and 4 month-old mice, respectively. Data represents mean±s.e.m. (unpaired t-test, t=(159)4.374). (c,d) Representative confocal images of Aβ halo (labelled with curcumin in c) and neuritic dystrophy (labelled with Lamp1 immunohistochemistry in d) in CRND8 mice. Scale bars, 5 μm in all panels. (e,f) Quantification of curcumin labelled protofibrillar Aβ halo (e) and Lamp1-labelled neuritic dystrophy area (f).N=62 plaques ineand 44 plaques inf. Data represents mean±s.e.m. (unpairedt-test,t=(60)5.508 foreand(40)2.404 forf) mo, months. Figure 8: Reduced microglia coverage in ageing is associated with an increased Aβ halo and neurotoxicity. ( a ) Quantification of microglia coverage (black bars) and microglia number (red bars) within 25 μm from the plaque edge at different ages in CRND8 mice. N >120 plaques from four mice per age group. Data represents mean±s.e.m. (unpaired t -test, t = (373) 3.905 and (286) 5.602 in microglia coverage and t = (286) 3.325 in microglia number). ( b ) Quantification of BrdU+ (5-bromodeoxyuridine ) microglia in 4 and 24 month-CRND8 mice. N=222 and 100 field of views analysed for 24 and 4 month-old mice, respectively. Data represents mean±s.e.m. (unpaired t-test, t=(159)4.374). ( c , d ) Representative confocal images of Aβ halo (labelled with curcumin in c) and neuritic dystrophy (labelled with Lamp1 immunohistochemistry in d) in CRND8 mice. Scale bars, 5 μm in all panels. ( e , f ) Quantification of curcumin labelled protofibrillar Aβ halo ( e ) and Lamp1-labelled neuritic dystrophy area ( f ). N =62 plaques in e and 44 plaques in f . Data represents mean±s.e.m. (unpaired t -test, t = (60) 5.508 for e and (40) 2.404 for f ) mo, months. Full size image Modulation of the microglia barrier ameliorates plaque neurotoxicity Given our evidence of greater dystrophic neuropathology near plaque microregions lacking microglia coverage and in aged mice with fewer microglia around plaques, we hypothesized that enhancing microglia coverage would have a neuroprotective effect. We have previously shown that microglia clustering around individual plaques can be manipulated by deletion of the chemokine receptor CX3CR1 (ref. 19 ). We thus crossbred CRND8 with CX3CR1 −/− mice and showed that CRND8/ CX3CR1 −/− mice had an increase in microglia process coverage of individual amyloid plaques ( Fig. 9a,b ). Furthermore, quantification of dystrophic neurites demonstrated that increased microglia process coverage in CRND8/ CX3CR1 −/− mice was associated with a significant reduction in neuritic dystrophy ( Fig. 9c ). A similar reduction in neuritic dystrophy following CX3CR1 knockdown was observed in another Aβ amyloidosis mouse model (5 × FAD; Supplementary Fig. 6 ). Interestingly, despite the fact that microglia coverage was increased in plaques of all sizes, we only observed reduced neuritic dystrophy in relatively small plaques, while larger ones, which are likely to be older [40] , had the same degree of dystrophy regardless of the CX3CR1 genotype ( Fig. 9c ). 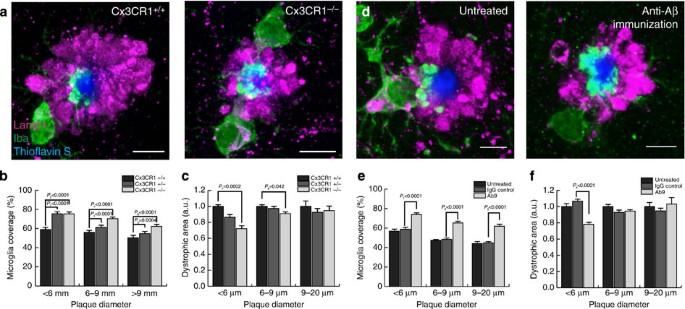Figure 9:CX3CR1deletion or Aβ immunization increases microglia coverage and reduces dystrophy. (a) Representative confocal images of microglia coverage and dystrophic neurites in 8month-CRND8 mice harbouring different copy numbers ofCX3CR1gene. (b) Quantification of microglia coverage as a function ofCX3CR1genotype and plaque size.t1=(140)7.465,t2=(159)8.939,t3=(202)5.890,t4=(249)13.28,t5=(56)3.760 andt6=(47)5.784. (c) Quantification of DN area as a function ofCX3CR1genotype and plaque size.t7=(170)3.828,t8=(256)2.047. (d) Representative confocal images of microglia coverage and dystrophic neurites in 4month-5 × FAD mice treated with passive anti Aβ immunization for 8 weeks. (e) Quantification of microglia coverage as a function of treatment and plaque size.t1=(324)8.093,t2=(385)15.59,t3=(66)5.848. (f) Quantification of DN area as a function of treatment and plaque size.t4=(218)4.557. For all quantifications data represents mean±s.e.m and compared using unpairedt-tests. In each genotype or treatmentN>3 animals and 40 plaques per animal. Scale bars, 5 μm in all panels. Figure 9: CX3CR1 deletion or Aβ immunization increases microglia coverage and reduces dystrophy. ( a ) Representative confocal images of microglia coverage and dystrophic neurites in 8month-CRND8 mice harbouring different copy numbers of CX3CR1 gene. ( b ) Quantification of microglia coverage as a function of CX3CR1 genotype and plaque size. t 1 = (140) 7.465, t 2 = (159) 8.939, t 3 = (202) 5.890, t 4 = (249) 13.28, t 5 = (56) 3.760 and t 6 = (47) 5.784. ( c ) Quantification of DN area as a function of CX3CR1 genotype and plaque size. t 7 = (170) 3.828, t 8 = (256) 2.047. ( d ) Representative confocal images of microglia coverage and dystrophic neurites in 4month-5 × FAD mice treated with passive anti Aβ immunization for 8 weeks. ( e ) Quantification of microglia coverage as a function of treatment and plaque size. t 1 = (324) 8.093, t 2 = (385) 15.59, t 3 = (66) 5.848. ( f ) Quantification of DN area as a function of treatment and plaque size. t 4 = (218) 4.557. For all quantifications data represents mean±s.e.m and compared using unpaired t -tests. In each genotype or treatment N >3 animals and 40 plaques per animal. Scale bars, 5 μm in all panels. Full size image We also tested passive anti-Aβ immunization as a method to enhance microglia process coverage given that anti-Aβ antibodies have been shown to induce microglia activation around plaques [29] , [30] . Indeed, administration of AB9 antibody to young 5 × FAD mice over 8 weeks induced a marked increase in microglia process coverage of fibrillar plaques ( Fig. 9d ). Similar to mice lacking CX3CR1 , the neuroprotective effect of increased microglia coverage was mainly observed in smaller plaques, which are likely to be the newest ones [40] ( Fig. 9e,f ). Taken together, we demonstrate that molecular manipulation of microglia can promote the barrier phenotype, which preferentially reduces local neurotoxicity around small early-stage plaques, suggesting that microglial processes wrapping the plaque core actively protect adjacent neurons from Aβ toxicity within a critical period during plaque development. We uncovered a previously unrecognized function of microglia in AD, which could be critical in the progression of amyloid deposition and its associated neurotoxicity. Our findings provide a framework for a better understanding of the role of microglia in neurodegeneration, which has gained significant importance as a result of evidence of genetic variants in microglia-related genes that increase the risk of late-onset AD [8] , [9] , [10] , [11] , [12] . Our data support a model in which microglia envelopment of amyloid plaques acts as a barrier that plays a critical role in modulating the degree of plaque compaction, a key factor in determining the ongoing affinity of plaques for soluble Aβ42 binding and consequent formation of protofibrillar Aβ42 hotspots. Several mechanisms could contribute to the microglia barrier function ( Supplementary Fig. 9 ). The close physical proximity of microglia processes, which are intertwined with the growing amyloid fibrils [21] , [22] , could act as a physical barrier that restricts their polymerization. Microglia processes create a crowded microenvironment that could prevent the normal outward elongation of the fibrils by promoting their bending or compaction [44] . In this scenario, microglia may insulate the growing fibril tips from recruiting interstitial soluble Aβ by promoting the formation of fibril conformers with reduced Aβ affinity [45] , [46] . The location of this physical barrier is relatively stable over months given the minimal motility of microglia process contacting the plaque compared with the highly motile processes away from the plaques ( Fig. 1 ). Nevertheless, our fluorescent Aβ42 sequential infusion over 60 days ( Supplementary Fig. 4 ) demonstrates a gradual shift in the hotspot location, likely due to the rearrangement of microglia processes. In addition to a physical cellular barrier, active microglia phagocytosis of oligomeric Aβ [7] , [19] and proteolytic activity by microglial secreted enzymes [47] , [48] could further reduce local polymerization and prevent fibril extension. The remarkable affinity to areas not covered by microglia processes of certain Aβ-binding dyes known to bind to protofibrillar Aβ, such as Curcumin [33] , [35] and THK-265, as well as exogenous soluble Aβ42, strongly support the concept that the microglia-uncovered areas are hotspots of active Aβ polymerization. The minimal Thioflavin-positive fibrils present in the hotspot region, is consistent with in vitro data demonstrating that low amounts of fibrils are necessary to efficiently polymerize oligomers and protofibrils from soluble monomers [49] . The fact that these small molecular weight dyes have very different binding properties compared with similarly sized Aβ- binding dyes derived from Congo red or Thioflavin-T ( Fig. 6 ), suggests that the high affinity for plaque areas of less compact amyloid in microglia-uncovered regions, is not due to the differences in molecular size of the ligand but rather specific biochemical affinities due to Aβ conformations. A similar phenomenon could explain the marked difference in the patterns of binding observed between Aβ40 and Aβ42. Currently, the Food and Drug Administration approved amyloid-binding positron emission tomography (PET) tracers used in patients with suspected AD, are derived from Thioflavin-T [50] and Stilbene [51] , which predominantly bind to the fibrillar plaque core and have negligible affinity for the protofibrillar Aβ42 around plaques. This could explain the poor correlation observed between PET signal and the degree of cognitive dysfunction when using these compounds for clinical imaging. The observation of a markedly greater protofibrillar Aβ halo and degree of neuritic dystrophy around fibrillar plaques of equal size when comparing young adults with ageing transgenic mice ( Fig. 8 ) further highlights the limitations of using PET tracers with affinity an for the plaque core. Our observation that the most toxic plaque areas are those that contain protofibrillar Aβ42 hotspots in microglia-uncovered regions, suggests that PET ligands with affinity to these areas could have a much greater specificity for clinical AD diagnosis and staging. Furthermore, similar molecules with specific affinity for the protofibrillar Aβ42 hotspots could be better at disrupting Aβ polymerization [52] , [53] than those that target the plaque core and may thus have greater therapeutic potential. Our findings that the overall degree of dystrophy around plaques is inversely correlated with the extent of microglia plaque envelopment, that areas covered by microglia processes have fewer dystrophic neurites and a lower rate of DN formation and that CX3CR1 knockdown and anti-Aβ immunotherapy reduce dystrophic neurites, strongly suggest that microglia exert a neuroprotective effect ( Supplementary Discussion ). Microglia, could act as a physical barrier that insulates plaques from their surrounding neurites, reducing their contact with potentially damaging Aβ protofibrils [54] , [55] . In addition, it has been shown in vitro that an increased ratio of Aβ42 to Aβ40 increases neurotoxicity [56] , [57] , [58] . This is consistent with our in vivo findings of hotspots of Aβ42 that co-localize with greater neuritic dystrophy. Furthermore, the active process of Aβ polymerization by itself could be more toxic than the static presence of fibrils [38] , [59] . Thus by creating a microenvironment that is not favourable to the ongoing Aβ42 polymerization, microglia could limit damage to the adjacent neurites. The role of microglia is further highlighted by our findings that in ageing, the decline in microglia proliferation [60] leads to a reduction in microglia numbers and degree of envelopment of amyloid plaques, which is associated with a dramatic increase in the size of the protofibrillar Aβ halo and in the number of dystrophic neurites. Thus, while microglia could cause secondary neurotoxicity due to their ability to secrete cytokines and reactive oxygen species [31] , it appears that in the vicinity of amyloid plaques where they can modulate the degree of amyloid compaction, they exert a net protective effect. Our observations could provide a mechanistic explanation for the increased plaque compaction and reduced neurotoxicity recently observed after manipulating IGF-1 (insulin like growth factor 1) signalling in AD mice [61] . It could also explain why despite equivalent fibrillar plaque load, greater oligomeric Aβ concentrations are predictive of the worse cognitive status in human patients [62] . Interestingly, we found that microglia envelopment was most effective at limiting protofibrillar Aβ accumulation and neuritic dystrophy around smaller plaques, even after CX3CR1 chemokine receptor deletion or anti-Aβ immunotherapy. This suggests that the importance of the microglia barrier is most prominent at the initial stages of fibrillar amyloid deposition and becomes less effective as plaques grow in size. This could explain why recent studies of microglia ablation in advanced stages of amyloidosis did not demonstrate any effect on plaque counts or neuritic dystrophy [63] . To what extent the microglia barrier plays a role in human AD remains to be determined. Given that in sporadic AD, the process of amyloid deposition is likely to be much slower than in transgenic models, it is possible that in human sporadic and familial AD, the microglia barrier would have unique spatial-temporal properties. Nevertheless, therapeutic interventions targeted at the microglia barrier may be most effective at the early stages of plaque evolution. However, the modest reduction of dystrophic neurites that we observed after anti-Aβ immunotherapy, despite a robust increase in the microglia envelopment, suggests that immunotherapy could have detrimental effects that counteract the beneficial effects of the microglia barrier. This could partly explain the failure of such therapeutic approach in clinical trials [27] , and suggests that a more specific strategy to enhance the microglia barrier may offer more effective neuroprotection. Together, our results demonstrate that microglia envelopment of amyloid plaques in AD is a highly coordinated process aimed at increasing the degree of compaction of fibrillar amyloid deposits while limiting the accumulation of potentially neurotoxic protofibrillar Aβ aggregates and shielding neurons from them. Understanding the precise mechanisms involved in this newly identified microglial function may further elucidate their neuroprotective role in AD and other neurodegenerative disorders. Transgenic mouse strains All animal experimental procedures were performed in accordance with the Federal and State regulations and approved by the Institutional Animal Care and Use Committee at Yale University and Northwestern University. Two AD mouse models were used in this study: CRND8 (Courtesy of Dr David Westaway, University of Toronto), which harbours human APP695 with KM670/671/NL (Swedish) and V717F (Indiana) mutations driven by the Prion promoter; and 5 × FAD (Courtesy of Dr Robert Vassar, Northwestern University), which overexpresses both human APP695 with KM670/671/NL (Swedish), V717I (London) and I716V (Florida) mutations and human PS1 harbouring M146L and L286V mutations under the Thy1 promoter. Heterozygous males were bred with C57Bl/6 females and litters were genotyped by PCR using the following primers: for CRND8 mice, 5′ primer:5′- AGGACTGACCACTCGACCAG-3′; 3′ primer: 5′-CGGGGGTCTAGTTCTGCAT-3′. For 5 × FAD mice, 5′ primer: 5′-AATAGAGAACGGCAGGAGCA-3′; 3′ primer: 5′-GCCATGAGGGCACTAATCAT-3′. Thy1-YFP mice were crossbred with AD mice, to visualize the dystrophic neurites around amyloid plaques in some experiments. To manipulate the CX3CR1 gene, mice with the CX3CR1 loci replaced by GFP ( CX3CR1 knock-in, The Jackson Laboratory 005582) were crossbred with CRND8 mice. Combined age-matched litters (6 months old unless otherwise indicated) were used for all experiments. Reagents and antibodies Fluorescently labelled Aβ peptides were provided by Anaspec (Hylite Fluor 555-Aβ42 60480-1, Hylite Fluor 488 labelled scrambled Aβ42 25382, Biotin-LC- Aβ42 24641-01, Hylite Fluor 488-Aβ40 60491-01 and Hylite Fluor 555-Aβ40 60492-01). Lyophilized peptides were dissolved in dimethylsulphoxide in a concentration of 1 mg ml −1 and stored as stock. Anti-Iba1 polyclonal antibody (Wako, 019-19741) was used to label microglia. Anti-GFAP polyclonal antibody (Dako, Z0334) was used to label astrocytes. Anti-Lamp1 (DSHB, 1D4B) and anti-Ubiquitin monoclonal antibody (Cell Signaling, 3936) were used to label dystrophic neurites. C-terminal specific antibodies for Aβ42 (Life technologies, 700254 and BioLegend, SIG39142-200) and Aβ40 (Millipore, AB5074P) were used for labelling amyloid plaques. 4G8 (BioLegend, SIG-39200) and MOAB-2 (Biosensis, M-1586-100), antibodies were used for labelling other Aβ fragments in the brain. Aβ conformation specific antibodies, A11 (Life Technologies, AHB0052) and OC (Millipore, AB2286), were used for labelling oligomeric Aβ. AlexaFluor-conjugated IgGs were used as secondary antibodies (Life technologies). Small molecule Aβ binding dyes used in the study are: FSB (Santa Cruz, sc-359845), Thioflavin S (Sigma-Aldrich, T1892), Thioflavin T (Sigma-Aldrich, T3516), Congo red (Sigma-Aldrich C6277), Thiazine red (MP Biochemicals, 05208297), Methoxy-X04 (gift from W. Klunk), BTA-1 (Sigma-Aldrich, B9934), Curcumin (Sigma-Aldrich, 08511) and THK-265 (Sigma-Aldrich, R277002). Recombinant adeno-associated virus (AAV) production DNA sequence of tdTomato fluorescent protein was ligated between the inverted terminal repea sites of an AAV packaging plasmid with CAG promoter and WPRE/SV40 sequence. HEK293T cells were co-transfected with this construct and a helper plasmid pDP2 (PlasmidFactory, #PF402) for 96 h and harvested. Virus was purified through iodixanol density centrifugation and titrated by infecting HEK293T cells. In vivo Aβ42 brain infusion via subarachnoid space Aβ peptide was injected into the mouse subarachnoid space as previously described [19] . In brief, mice were anaesthetized with ketamine-xylazine, a thin-skull window about 1 mm in diameter was made with a dental drill at 5.0 mm anteroposterior, 2.5 mm mediolateral from bregma. A ~300 μm × 300 μm piece of skull was lifted with a 25 G needle to expose the tissue underneath, and the dura was carefully removed without touching the brain parenchyma. Aβ peptide was diluted in fresh sterile artificial cerebrospinal fluid (ACSF) (1:9 v/v) at 37 °C for 10 min before placing on ice. The solution was filled into a Tygon tube connected to a polypropylene tip with an outer diameter of 70 μm. A programmable syringe pump with a Hamilton syringe was connected to the tube. The tip was then inserted into the exposed subarachnoid space and fixed with cyanoacrylate glue. 10 μl of the Aβ solution was injected at speed of 0.2 μl per min. After injection, the tip was removed and the mouse scalp was sutured. Mice were put on a heating pad for recovery and received Buprenex analgesia. At various time points after injection, mice were either imaged in vivo with two-photon microscopy or killed for fixed tissue confocal imaging. Fresh brain slice Aβ labelling Mice were decapitated under anaesthesia. The brains were dissociated on cooled ACSF with continuous oxygenation. After dissociation, the brains were immediately transferred onto a vibratome. Coronal sections were made at 150-μm thickness. Fluorescently labelled Aβ42 was added into the incubation bath to make a final concentration of 2 μg ml −1 . Slices were incubated on a shaker for 1 h at 4 °C and then washed twice with ACSF. After the last wash, slices were fixed in 4% paraformaldehyde at room temperature for 1 h. Fixed slices were then washed with PBS before imaging. Fixed brain slice Aβ labelling Fixed brain slices were washed three times with PBS, then incubated at 95 °C for 30 min (buffer: 10 mM sodium citrate, 0.05% Tween-20 (v/v)). Slices were further washed in PBS with 0.2% Triton-X100 before adding fluorescently labelled Aβ to a final concentration of 5 μg ml −1 . Slices were incubated at 4 °C on a shaker for 24 h and then washed three times in PBS before mounting for imaging. Immunohistochemistry The fixed brains were sectioned to 30-μm thickness using a Leica vibratome (VT1000S). For ubiquitin, sections underwent heat-induced antigen retrieval at 95 °C for 30 min (buffer: 10 mM sodium citrate, 0.05% Tween-20 (v/v), pH=6.0). For Aβ-antibody staining, sections were pretreated with an antigen retrieval buffer containing 70% formic acid in 1 × PBS for 10 min and washed with 1 × PBS. Primary antibodies were diluted in saline with 0.2% (v/v) Triton-X100 and 4% (v/v) normal goat serum (Jackson ImmunoResearch 005-000-121). The sections were incubated with the primary antibody solution at 4 °C for 2 days followed by secondary antibodies for 5 h. For amyloid plaque staining, a TS solution (0.0003% (m/m)) was used for a 15-min incubation at room temperature. Stained sections were mounted onto glass slides with PermaFluor mounting medium (Thermo Scientific, TA-030-FM). Quantitative analysis of Aβ42 hotspots in fixed brain slices Aβ labelling was visualized with a Leica SP5 laser scanning confocal microscope with a Leica 63 × oil objective (N.A 1.4). Images were taken with a standard step size of 0.7 μm. Emission of TS and fluorescently labelled Aβ were collected sequentially. All images were taken with a 512 × 512 pixel resolution and 8-bit colour depth. All images were processed using custom-written ImageJ macros. A maximum intensity Z -projection of five optical slices through the centre of the plaque was made to create a single image for analysis. Plaque area was determined by setting a threshold of 3 s.d. above the entire image mean intensity. For analysing the interface between plaque and hotspots, the selection of thresholded plaque area was enlarged 2μm radially outward to include the hotspot area. Fluorescence intensities in both the channels were analysed along a line between the centre point of the plaque and each individual point in the perimeter of the enlarged selection. Fluorescent intensities were normalized to a 0–1 scale with the highest pixel intensity of the image as 1. To calculate the slope of fluorescent intensity change, a linear regression was fitted to the data set 10 points before and after the thresholded plaque border. To calculate the total fluorescence in the plaque halo (the area under the curve), sum of pixel intensities within the thresholded plaque border was used. Each line was categorized as hotspot or non-hotspot based on its maximum intensity in the Aβ42 channel and as microglia-covered or -uncovered based on its microglia intensity (as in Supplementary Fig. 3 ). For the purpose of display, each line was resampled into 50 points using ‘Array.resample’ function in ImageJ. Microglia coverage and DN quantification Imaging conditions were the same as described above except for having three emission channels. Plaques were chosen from cortex, layer IV–VI. Images were numbered randomly and blinded for analysis. All images were processed with a customized ImageJ macro. Plaque area was identified by setting the threshold for 1 s.d. above the entire image mean intensity. Five optical slices through the centre of the plaque were used for analysis. On each slice, the intersection between the tips of microglia process and the plaque perimeter were identified manually. The proportion of the plaque perimeter covered by microglia processes was calculated by summing the arcs of plaque perimeter that co-localized with microglia processes. DN area was determined by setting a threshold for 1 s.d. above the entire image mean intensity. The plaque area was excluded from this area quantification. In the experiment using Thy1-YFP mice, dystrophic neurites were counted manually. To compare the area with or without microglia coverage, the coverage angle was converted to a triangular selection. The selection was then extended to the limits of the image. The overlap between this extended selection and the dystrophic area was defined as the dystrophic area in the covered region of the plaque. DN area was normalized per angular degrees of associated plaque perimeter. That is, the DN area was divided by the relative amount of the plaque covered or uncovered in angular degrees using the formulas below: (1) for microglia-covered areas: Dystrophy/coverage=(area of dystrophic neurites outward of microglia-covered plaque perimeter)/(degrees of arc of microglia coverage). (2) for microglia-uncovered areas: Dystrophy/coverage=(total area of dystrophic neurites—covered portion of DN area)/(360-arc of microglia coverage). A similar analysis was used for comparing the dystrophic neurites count, Aβ42 binding, curcumin and THK265 fluorescence. Plaques with diameter between 6 to 9 μm were used in these analyses. For each measurement, the average of the results for five optical slices was reported as a measurement for individual plaque. Statistical analyses were performed in GraphPad Prism, using two-tailed t -test assuming same s.d. In vivo two-photon time-lapse imaging of Aβ binding Mice received FSB injection (intraperitoneal (i.p.) 7.5 mg kg−1) 2 days before the experiment. In the experiments requiring astrocyte labelling, freshly-made sulforhodamine 101 solution (5 mM, 100 μl per mouse) was injected (I.V.) 1 day before the experiment. Mice were anaesthetized with ketamine-xylazine, a thin-skull window about 2 mm in diameter was made with a dental drill at 2.0 mm anteroposterior, 3 mm mediolateral from bregma. A 200 μm × 200 μm opening on the posterior side of the window was made with a 25 G needle to expose the tissue underneath. And then the dura was carefully removed. Using a motorized manipulator (Sutter instrument, MP-285), a micro glass-pipette filled with Aβ peptide solution (described above) was inserted into the opening. The pipette was connected with a picospritzer microinjection system (Parker Hannifin Corporation, 051-0500-900) set at 30 psi. Infusion of Aβ solution was initiated by giving several 100-ms pulses through the picospritzer. In vivo two-photon imaging (Prairie technology) was performed with a Ti-Sapphire laser (Mai Tai Spectra Physics) with a 20 × water immersion objective (Leica, NA 1.0). Time-lapse images were taken ~200 μm away from the pipette tip. To increase the probability of capturing the binding process, XYZT stacks were taken from a 100 μm (X, 512 pixel) × 100 μm (Y, 512 pixel) × 50 μm ( Z , step size 3) volume. Each XYZ cycle took about 20 s. Aβ42-555, Aβ42-488 and GFP fluorophores were excited at 925 nm; FSB and sulforhodamine 101 were excited at 850 nm. To analyse Aβ binding, images were first corrected for minor movement artifacts using ‘StackReg’ plugin in Fiji ( www.fiji.sc ). Subsequently different channels were merged together using the ‘Merge Channels…’ function. Each region for analysis was extracted from the original XYZT stack by making a three optical slices projection centred at the middle plane of the amyloid plaque. In the projected XYT stacks, plaque regions were defined by thresholding the FSB channel (3 s.d. from the mean). Microglia regions were defined by thresholding the GFP channel (1.5 s.d. from the mean) and excluding the plaque regions. Aβ42 binding was reported as ratios of fluorescence intensity between the red channels (Aβ42-555) and the green channels ( CX3CR1 -GFP) to account for the change of focal plane. Short-term in vivo two-photon imaging of microglia dynamism Microglia were labelled by crossing CRND8 or 5 × FAD mice with CX3CR1 -GFP mice. 8–10 month- old mice were used in these experiments. Mice were anaesthetized with ketamine-xylazine, a craniotomy window about 2 mm in diameter was made at 3.0 mm anteroposterior, 3 mm mediolateral from bregma. The duramater was removed with a #7 tweezer (Dumont) avoiding bleeding or damage to the cortex. Topical application of thiazine red solution was used to label amyloid plaques for 30 min. A thin glass coverslip (#0) was pre-cut and fixed directly on the skull after the excess dye was washed out. In vivo two-photon microscopy imaging was performed. XYZT stacks were taken from a 200 μm (X, 1024 pixel) × 200 μm (Y, 1024 pixel) × 100 μm ( Z , step size 3) volume. GFP and Thiazine red were excited at 900 nm.To analyse microglia process dynamism, images were first corrected for minor movement artifacts using ‘StackReg’ plugin in Fiji. Each region for analysis was extracted from the original XYZT stack by making a three optical slice projection centred at the middle plane of the amyloid plaque. In the projected XYT stacks, plaque regions were defined by thresholding the FSB channel (3 s.d. from the mean). Microglia regions were defined by thresholding the GFP channel (1.5 s.d. from the mean). Dynamism was determined by calculating the overlap between the thresholded areas of microglia processes between the first time point and later time points. Long-term in vivo two-photon imaging of microglia dynamism Microglia were labelled by crossing CRND8 with CX3CR1 -GFP mice. Mice that were 10–12 months old were used in these experiments. Mice were injected with FSB (7.5 mg kg −1 , i.p.) 2 days before each imaging session. In the first session, a thin-skull window about 2 mm in diameter was made with a dental drill at 2.0 mm anteroposterior, 3 mm mediolateral from bregma. The window was polished before imaging in the subsequent sessions with a micro blade (Surgistar, 6961). A landmark picture was taken of the surface pial vessels. All coordinates of imaging regions relative to the landmark location were recorded. In later imaging sessions, relocation was achieved by matching the landmark blood vessel shape and orientations to the original landmark picture and then reloading the coordinates. In each plaque region, XYZ stacks were taken from a 150 μm (X, 1024 pixel) × 150 μm (Y, 1024 pixel) × 30 μm ( Z , step size 1) volume. GFP was excited with 950 nm laser and FSB was excited with 850 nm laser. To analyse microglia process dynamism, the GFP and FSB channels were first merged together using the ‘Merge Channels…’ function. Each region for analysis was extracted from the original XYZ stack by making a three optical slices projection centred at the middle plane of the amyloid plaque. The projected images from the same location at the different time points were aligned manually based on maximizing the overlap of the plaque centre, microglia cell bodies and lipofuscin granules. After alignment, pictures from the same location were compiled into a single stack. In each slice of the stack, the plaque regions were defined by thresholding the FSB channel (3 s.d. from the mean). The intersection between the tips of microglia process and the plaque perimeter were identified manually. The plaque perimeter was divided into 360° based on the angle from the plaque centre and coverage was calculated using the summed degrees of plaque perimenter arcs that co-localized with microglia processes. These coverage data was recorded as a 360 length binary array for each time point. In all the time series, the first imaging session was used as the reference and designated as ‘day0’. Stable processes were calculated by multiplying the array from day 0 to day 1, 5, 10 and 50. Added processes were calculated by subtracting the stable processes from day 1, 5, 10 and 50’s arrays. In vivo two-photon imaging of DN turnover CRND8 and 5 × FAD mice were crossbred with CX3CR1-GFP mice to visualize microglia. To label dystrophic neurites the mice were either further crossbred with Thy1-YFP mice or injected with AAV-tdTomato virus through the subarachnoid space as described above. Mice were injected with FSB, i.p. (7.5 mg kg −1 ) 1 day prior to the first imaging session to label amyloid plaques. Mice were anaesthetized with Ketamine/Xylazine. A thinned-skull window ~500 μm in diameter was made at −2 mm to bregma and 2.5 mm lateral to the midline. In vivo two-photon imaging was performed as described above. Amyloid plaques were identified within 150 μm of the pial surface. Individual amyloid plaques were imaged with 825 nm excitation for FSB and 950 nm excitation for both microglia (GFP) and DNs (YFP or tdTomato). Image stacks were taken for each plaque at a 1-μm step size. Plaque location was recorded and each plaque was relocated 5 days later and imaged under the same conditions. For analysis, a maximum intensity Z -projection of three optical slices at the plaque centre was made. Microglia coverage was determined as described above. DN formation and elimination events were identified based on appearance or disappearance of DN in the second time point. Events were counted manually and categorized based on their proximity to microglia-covered and uncovered plaque areas. The probability of elimination was calculated as the number of elimination events/number of pre-existing DNs. The probability of formation was calculated as the number of events in microglia-covered or -uncovered regions/arc in degrees of microglia-covered or -uncovered plaque perimeter. Passive immunization treatment Ab9 administration was done as previously described [30] . In brief, 6-week-old 5 × FAD mice were randomly divided into three groups. One group received no injection. The second group received i.p. injection of 1 mg ml −1 mouse control IgG every 2 weeks. The third group received i.p. injection of 1 mg ml −1 Ab9 antibody every 2 weeks. One week after the fourth injection, mice were killed and the brains were collected for quantitative immunohistochemistry. Statistics Data are represented as mean±s.e.m. Histogram plots were used to observe the approximate Gaussian distributions, upon which two-tail unpaired Student’s t -tests were employed for comparisons between the two groups. A probability of P <0.05 was considered indicative of the significant differences between the groups. Data were additionally normalized to the average value of the measurements in the control group for better scaling of the result. In the experiments with CX3CR1 gene knockout and Aβ passive immunization, we report statistical comparisons using both plaque numbers ( Fig. 9 ) and animal numbers ( Supplementary Fig. 7 ). Regardless of the method used, the results are equivalent in magnitude and statistically significant. How to cite this article: Condello, C. et al. Microglia constitute a barrier that prevents neurotoxic protofibrillar Aβ42 hotspots around plaques. Nat. Commun. 6:6176 doi: 10.1038/ncomms7176 (2015).